Controlling the direction of rectification in a molecular diode A challenge in molecular electronics is to control the strength of the molecule–electrode coupling to optimize device performance. Here we show that non-covalent contacts between the active molecular component (in this case, ferrocenyl of a ferrocenyl–alkanethiol self-assembled monolayer (SAM)) and the electrodes allow for robust coupling with minimal energy broadening of the molecular level, precisely what is required to maximize the rectification ratio of a molecular diode. In contrast, strong chemisorbed contacts through the ferrocenyl result in large energy broadening, leakage currents and poor device performance. By gradually shifting the ferrocenyl from the top to the bottom of the SAM, we map the shape of the electrostatic potential profile across the molecules and we are able to control the direction of rectification by tuning the ferrocenyl–electrode coupling parameters. Our demonstrated control of the molecule–electrode coupling is important for rational design of materials that rely on charge transport across organic–inorganic interfaces. Optimizing the performance of organic and molecular electronic devices has been a major challenge because of a poor understanding of the organic–electrode interfaces [1] , [2] , [3] , [4] , [5] , [6] , [7] . Coupling the molecular frontier orbital to one electrode (or both) is key to generate electronic function with optimal device performance for a range of applications including molecular-based rectification, spin-transport and memory [8] , [9] , [10] , [11] , [12] . Strong electronic coupling ensures that the molecular frontier orbital efficiently follows the Fermi level of the electrode to which it is coupled under bias, but it results in hybridization of orbitals and in a corresponding broadening of the molecular energy levels and large leakage currents [8] . On the other hand, weak electronic coupling minimizes hybridization, ensuring narrow molecular energy levels, but the molecular orbitals cannot follow the Fermi levels of either electrode, hampering electronic function [8] . Hence, many applications require coupling that is strong enough to control electronic function but with the molecular orbitals localized in the molecule. Here we show that we turned around a molecular diode with good performance (with high rectification ratios of up to 85) by fine-tuning the interactions between the active component of the diode and the electrodes, ensuring narrow molecular energy levels and small leakage currents. Non-covalent molecule–electrode interactions can be strong enough to form metal–molecule–metal junctions [13] , [14] , [15] , but have only rarely been identified to have a crucial role in generating electronic function. For example, Meisner et al . [16] showed that these interactions can be used to generate a ‘molecular potentiometer’, and Díez-Pérez et al . [6] showed that non-covalent interactions can be used to control the conductance across single molecules. In this article, we show that non-covalent coupling between the active component of the molecule (that is, ferrocenyl (Fc)) and the electrode allows for the molecular frontier orbital (here the highest occupied molecular orbital (HOMO) located at the Fc) to follow changes in the Fermi level of the electrode it is interacting with. By placing the Fc units at 14 different positions within the alkyl chain of the self-assembled monolayers (SAMs) of the form SC n FcC 13− n (C n is the number of aliphatic carbons (CH 2 or a terminal CH 3 ) with n =0 to 13), we control the direction of rectification and determined the optimal Fc–electrode coupling experimentally by varying n . From our experiments, we conclude that non-covalent coupling can be strong enough to induce electronic function, that is, rectification, but with sufficiently narrow molecular energy levels to obtain good electronic performance, that is, high rectification ratios. In addition, by examining the rectification ratio as a function of the Fc position within the SAM, we find that the shape of the electrostatic potential profile is nonlinear, which is likely due to a screening of the electric field in the junction by the molecule. We believe that our findings are helpful in the future design of other types of (bio)molecular- and organic-electronic devices. The molecular diodes Previously, we have reported on the mechanism of charge transfer across molecular diodes with SAMs of SC 11 Fc on ultra-flat template-stripped silver-bottom electrodes (Ag TS ; henceforth left electrode) and EGaIn top electrodes (henceforth right electrode; a non-Newtonian liquid–metal alloy of eutectic In and Ga) [17] , [18] , [19] , including temperature-dependent J (V) measurements [20] (others have studied the mechanism rectification of SC n Fc SAMs in other types of junctions [21] , [22] , [23] ). This so-called ‘EGaIn’ technique is well established [24] , [25] , [26] , [27] and has been used in a wide range of physical–organic studies [20] , [28] , [29] , [30] , [31] , [32] , [33] . The HOMO is located at the Fc unit, which is separated from the left electrode by the alkyl chain (similar to the junction schematically shown in Fig. 1c for a SAM of SC 13 Fc) and in non-covalent contact with the right electrode. At forward bias (positive voltage in the right electrode), the HOMO (which follows the right electrode) falls in between the energy window defined by the electrodes’s Fermi levels and participates in the charge transport mechanism, resulting in sequential tunnelling (with an activation energy of 77±5 mV), that is, the diodes are in the ‘on’ state and allow current to pass through the junction. At opposite bias (negative voltage in the right electrode), the HOMO falls below both Fermi levels and cannot participate in the transport, resulting in a one-step electrode-to-electrode direct tunnelling process, that is, the diodes are in the ‘off’ state and block the current, leaving just a small ‘leakage current’ (as indicated in Fig. 1d ). This change in the mechanism of charge transport effectively reduces the width of the tunnelling barrier in only one direction of bias, resulting in rectification ratios R ≡ | J (−1.0 V)/ J (+1.0 V)| as large as ~1.0 × 10 2 (ref. 20 ). This definition of R implies that the junctions allow the current to pass through at negative bias when R >1 or at positive bias when R <1. 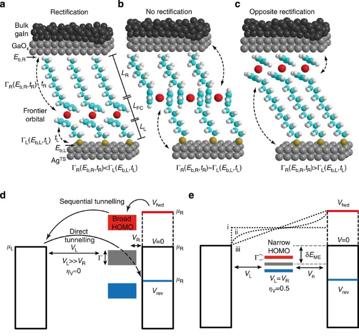Figure 1: The junctions of the form AgTS-SCnFcC13−n//Ga2O3/EGaIn. Idealized schematic illustrations of the junctions with the Fc units in non-covalent contact with the bottom electrode defined as the left electrode (n=3,a), in the middle of the junction (n=6,b), and in non-covalent contact with the top electrode, defined as the right electrode (n=13,c). The schematics illustrate how the spatial disposition of the HOMO level (which is centred on the Fc unit) with respect to the electrodes can be controlled as a function ofn(the alkyl linkers are flexible and the average Fc–electrode distances are given inFigs 3and5). The Fc unit couples to the electrodes as indicated by the dashed arrows. For more realistic images of the structures of the SAMs, we refer to structures obtained from molecular dynamics simulations (Fig. 3). The corresponding energy level diagrams for coupling with large (d) and minimal (e) molecular frontier orbital broadening. The curved arrows indindicate the bias-dependent change in the mechanism of charge transport from direct to sequential tunnelling as explained in the text. The various coupling parameters that control device performance are defined in the text. The dotted lines ineindicate schematically the flat (i) and ramp-like (ii, iii) electrostatic potential profiles. Figure 1: The junctions of the form Ag TS -SC n FcC 13− n //Ga 2 O 3 /EGaIn. Idealized schematic illustrations of the junctions with the Fc units in non-covalent contact with the bottom electrode defined as the left electrode ( n =3, a ), in the middle of the junction ( n =6, b ), and in non-covalent contact with the top electrode, defined as the right electrode ( n =13, c ). The schematics illustrate how the spatial disposition of the HOMO level (which is centred on the Fc unit) with respect to the electrodes can be controlled as a function of n (the alkyl linkers are flexible and the average Fc–electrode distances are given in Figs 3 and 5 ). The Fc unit couples to the electrodes as indicated by the dashed arrows. For more realistic images of the structures of the SAMs, we refer to structures obtained from molecular dynamics simulations ( Fig. 3 ). The corresponding energy level diagrams for coupling with large ( d ) and minimal ( e ) molecular frontier orbital broadening. The curved arrows in d indicate the bias-dependent change in the mechanism of charge transport from direct to sequential tunnelling as explained in the text. The various coupling parameters that control device performance are defined in the text. The dotted lines in e indicate schematically the flat (i) and ramp-like (ii, iii) electrostatic potential profiles. Full size image For the present study, we formed junctions with a series of 14 SAMs, namely SC n FcC 13− n (with n =0–13) on Ag TS and Au TS electrodes. Figure 1a–c show schematically the junctions for SAMs with n =3, 6 and 13, and illustrates how the position of the Fc units (at which the HOMO of the molecule is located) in the SAM can be controlled by simply changing the lengths of the ‘insulating’ alkyl chains L L and L R , which, in turn, determine the nature and strength of the Fc–electrode interaction (as described in the section ‘Coupling parameters’ below). We choose this system because our previous studies of similar SAMs (that is, SC 11 Fc) [17] , [18] , [19] , [20] show that these junctions perform well (the value R of 1.0 × 10 2 is large enough for physical–organic studies of charge transport) and the mechanism of rectification has been studied in a broad range of temperatures [20] , making this a good platform to demonstrate reversal of the rectification at the molecular level and to study the Fc–electrode coupling in more detail. We use the data to qualitatively describe for the first time the shape of the electrostatic potential profile purely on the basis of experimental measurements. Coupling parameters Figure 1 shows the various coupling parameters and the shapes of the possible electrostatic potential profiles of molecules sandwiched between electrodes. Following the narrative put forward by Moth-Poulsen and Bjørnholm [8] , the degree of electronic coupling of a molecular orbital with an electrode is normally expressed in terms of an energy coupling parameter Γ i (eV), which often depends on the strength of the bond of the molecule with the electrode i , the binding energy E b,i (here the metal–thiolate bond or the non-covalent SAM–top electrode contact), and on the coupling between the electrode and the molecular frontier orbital, t i (here the Fc–electrode interactions). The total electronic coupling strength of the HOMO to the two electrodes is then Γ=Γ R ( E b,R , t R )+Γ L ( E b,L , t L ), which in turn defines the broadening of the HOMO energy level [12] , [34] , [35] . Note that even in the case where the binding energies are large, the HOMO can still be narrow when placed sufficiently far away from the electrodes, since the t L and t R decay exponentially with the respective Fc–electrode distances L L and L R (which are related to n ). Importantly, Γ R and Γ L determine the rate at which the electron tunnels into and out of the molecule in a sequential tunnelling process. At sufficiently high temperatures (for example, above ~150 K for SC 11 Fc [20] ), the conduction becomes thermally assisted, involving intramolecular relaxation processes of the Fc and leading to larger tunnelling rates. This is most likely the case of the experiments presented here (conducted at room temperature), therefore Γ R and Γ L effectively describe a thermally assisted sequential tunnelling conduction process (detailed temperature-dependent data will be published separately). In all our junctions, the SAMs are chemisorbed to the bottom(left) electrode via a metal–thiolate bond (with typical binding energies of 1–2 eV) while the top(right) electrode forms a non-covalent contact with the SAMs (with correspondingly low energies). We hypothesize that the values of E b,R and E b,L are independent of n , but t R and t L depend on n . As shown below in the section ‘The molecule–electrode interaction’, this hypothesis holds for n =3–13, but for values of n <3 the strong electrode–Fc interaction results in hybridization of the HOMO with the orbitals of the bottom(left) electrode. In principle, rectification can occur when E b,L ≠ E b,R , but it has been shown experimentally that varying the nature of the metal–molecule interaction only results in modest rectification ratios, for example, R <3.5 (refs 36 , 37 ). Our junctions only barely rectify ( R <2) when the Fc units are in the middle of the junctions, or when the Fc is absent, that is, junctions with n-alkanethiolate SAMs [18] , [19] , [20] . The spatial position of the Fc with respect to the electrodes is related to the lengths of both alkyl chains L L and L R , as shown in Fig. 1a , and determines the potential drops at both sides of the Fc ( V L and V R ). Correspondingly, the junctions are also electrically asymmetric when L L ≠ L R . This asymmetry is given by the dimensionless division parameter η V = V R /( V L + V R ), which gives the ratio of the voltage drop between the molecule and the right electrode [34] , [38] . In principle, rectification can only occur when η V ≠½, that is, when the junction is asymmetric and the Fc units are close to the left or right electrodes. By varying the value of n we can control the spatial position of the Fc relative to both electrodes and consequently control η V between 0 and 1, that is, change the direction of rectification. As shown in the next section, we can indeed control the value of η V between ~0 and 1 and turn around a diode at the molecular level. Small values of δ E ME (the offset in energy between the HOMO and the Fermi level it is coupled to; see Fig. 1 ) [12] result in low turn-on voltages at forward bias ( V fwd ), but also in large leakage currents of the diodes in the off state, as the HOMO can fall in the energy window between the two Fermi levels at relatively low reverse bias ( V rev ). This effect becomes important when Γ is comparable to δ E ME . On the contrary, for large values of δ E ME , the HOMO cannot participate in the mechanism of charge transport within the applied bias window and the diodes cannot rectify. In principle, to ensure optimal diode behaviour, the Fc–electrode coupling strength has to be fine-tuned while keeping η V close to 1 or 0, and δ E ME moderate to minimize leakage currents. In the section ‘The molecule–electrode interaction’, we show that this condition can be met in our junctions, with a HOMO level sufficiently narrow and a large enough δ E ME to ensure good diode performance, when n =3 or n ≥11. The electrostatic potential profile can be either flat or ramp-like (i and ii–iii in Fig. 1e , respectively), but it has not been measured directly in experiments so far. A departure from linear behaviour is commonly ascribed to a screening of the electric field by the molecules, and its expected features have been well described theoretically [39] , [40] , [41] , [42] , [43] . The shape of the electrostatic potential profile can be qualitatively determined by examining the dependence of R on n as the value of R depends on η V , which, in turn, depends on V L and V R along L L and L R , respectively. Following this assumption, in the section ‘The mechanism of rectification’, we qualitatively discuss the shape of the electrostatic potential profile in our SAM-based junctions. 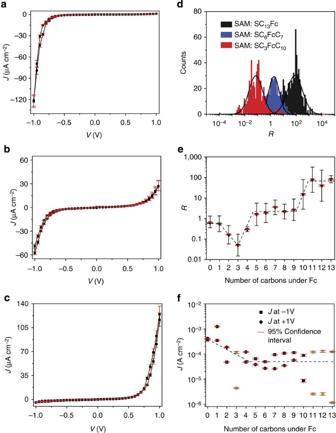Figure 2: The electrical charactistics of the tunnelling junctions. AverageJ(V) curves of junctions with SAMs of SC13Fc (a), SC6FcC7(b) and SC3FcC10(c). SeeSupplementary Figs 4 and 5,Supplementary Table 2andSupplementary Methods: ‘Statistical analysis’ for all SAMs with log-standard deviations, details of the statistical analysis and histograms of the current densities. (d) Histograms of the rectification ratios of these junctions with Gaussian fits to the histograms. (e) The rectification ratio as a function ofn. The error bars indicate one log-standard deviation (black bar) or 95% confidence level intervals (red bar). The dashed line is a guide to the eye. (f) The current density measured at −1.0 V and +1.0 V as a function ofn. The dashed line indicates the regimes in which the diodes are in the on-state. The diode in the off state are at negative bias only forn=3, whereas only forn>10, the diodes are in the off state at positive bias; these most efficient diodes are indicated in green. Charge transport and SAM structure Figure 2a–c shows the J (V) curves of the junctions − J is the current density (A cm −2 ) and V is the applied bias (V)—with SAMs of SC n FcC 13− n with n =3, 6 and 13, and Fig. 2d shows the corresponding histograms of the values of R measured at ±1.0 V (see Supplementary Figs 4 and 5 for all data). These J (V) curves represent averages determined using large data sets (~500 traces for each type of junction) with an average yield in non-shorting junctions of 91% ( Supplementary Table 2 ). The data clearly show a control of the electrical characteristics of the junctions and demonstrate the reversal of the direction of rectification for different positions of the Fc unit within the junction. Figure 2e shows the nonlinear change in rectification as the position of the Fc unit is adjusted within the SAM, and provides four important observations. First, the rectification is low ( R is close to unity) when the Fc units are close to the left electrode ( n <2). Second, the rectification increases substantially reaching a value of R of ~0.052 for n =3 but decreases abruptly again as the Fc units are placed further away from the left electrode ( n =4 and 5). The rectification remains low and almost constant ( R ~2) when the Fc is roughly equidistant from both electrodes (5≤ n ≤9). Finally, the rectification increases abruptly saturating above n =11 at a high value ( R ~80) when the Fc units get within five carbons from the right electrode ( n >9). Figure 2f shows the current densities as a function of n , from which we conclude that the diodes that do not rectify are always in the on-state, allowing current to flow at both negative and positive bias. Figure 2: The electrical charactistics of the tunnelling junctions. Average J (V) curves of junctions with SAMs of SC 13 Fc ( a ), SC 6 FcC 7 ( b ) and SC 3 FcC 10 ( c ). See Supplementary Figs 4 and 5 , Supplementary Table 2 and Supplementary Methods : ‘Statistical analysis’ for all SAMs with log-standard deviations, details of the statistical analysis and histograms of the current densities. ( d ) Histograms of the rectification ratios of these junctions with Gaussian fits to the histograms. ( e ) The rectification ratio as a function of n . The error bars indicate one log-standard deviation (black bar) or 95% confidence level intervals (red bar). The dashed line is a guide to the eye. ( f ) The current density measured at −1.0 V and +1.0 V as a function of n . The dashed line indicates the regimes in which the diodes are in the on-state. The diode in the off state are at negative bias only for n =3, whereas only for n >10, the diodes are in the off state at positive bias; these most efficient diodes are indicated in green. Full size image To relate the electrical characteristics of the junctions to the SAMs, we characterized the supramolecular structures of the SAMs and made the following observations ( Fig. 3 ). The good agreement between the Fc unit orientations obtained by near-edge X-ray absorption fine structure spectroscopy (NEXAFS; see Supplementary Fig. 7 and 8 ) and molecular dynamics simulations (MD) indicates that the MD models provide a reliable description of the SAM structures ( Fig. 3a–d ). The angle-resolved X-ray photoelectron spectroscopy (ARXPS) and MD data (see Supplementary Fig. 15 ) are in good agreement and show near-Ångström precision placement of the Fc unit within the SAM. Note that the thickness of the SAM decreases slightly when decreasing the value of n from 1.8 to 1.4 Å ( Fig. 3e ), due to more crumpled packing of alkyl groups above the Fc when compared with the alkyls below the Fc (see Supplementary Fig. 16 ). Finally, the cyclic voltammetry data (see Fig. 3f and Supplementary Figs 1 and 2 ) and XPS data show that the SAMs with n <3 have shorter substrate-to-Fc distances and lower surface coverages than expected from MD. These discrepancies between molecular dynamics and experiment are due to an underestimation of the Fc–electrode interaction for n <3, and are reconciled using quantum mechanical calculations (for details, see Methods). The resulting loose packing of the SAMs for n <3 caused an increase in the currents measured at ±1.0 V ( Fig. 2f ), but the yields in working devices were nearly the same (86–100%) over the entire range of values of n ( Supplementary Table 2 ). 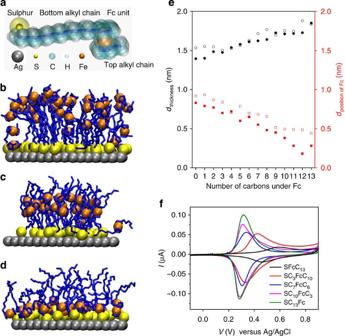Figure 3: Structural characterization of the SAMs on AgTSand AuTSsurfaces. (a) The molecular structure of S(CH2)12FcCH3, one of the SCnFcC13−nseries of molecules. In this case, the bottom alkyl chain below Fc is (CH2)12and the top alkyl above Fc is CH3. Side-views of representative structures of the SC12FcC1(b), SC7FcC6(c) and SFcC13SAMs (d) on silver obtained by molecular dynamics. The full models (containing >1,000 molecules and including SAMs on both Ag and Au) are shown inSupplementary Fig. 14. (e) The film thicknesses and position of the iron atom below vacuum within the SAMs on AuTSdetermined from ARXPS (seeSupplementary Fig. 6for the XPS spectra) and molecular dynamics as a function ofn, that is, the number of carbons under the Fc moiety (for details seeSupplementary Methods: ‘Molecular Dynamics simulations: Model details and simulation protocol’). Error bars on the time- and structure-averaged MD data are 0.2–0.4 nm. (f) Cyclic voltammograms of SAMs of SCnFcC13−non Au withn=0, 3, 7, 10 and 13 (seeSupplementary Figure 1for cyclic voltammograms for all SAMs) recorded at a scan rate of 1.0 V s−1with aqueous 1.0 M HClO4as the electrolyte solution. The peak oxidation potentials of the SAMs on AuTSgenerally increase with decreasingnsuggesting the alkyl chains above the Fc units effectively shield the Fc units from the electrolyte solution. Figure 3: Structural characterization of the SAMs on Ag TS and Au TS surfaces. ( a ) The molecular structure of S(CH 2 ) 12 FcCH 3 , one of the SC n FcC 13−n series of molecules. In this case, the bottom alkyl chain below Fc is (CH 2 ) 12 and the top alkyl above Fc is CH 3 . Side-views of representative structures of the SC 12 FcC 1 ( b ), SC 7 FcC 6 ( c ) and SFcC 13 SAMs ( d ) on silver obtained by molecular dynamics. The full models (containing >1,000 molecules and including SAMs on both Ag and Au) are shown in Supplementary Fig. 14 . ( e ) The film thicknesses and position of the iron atom below vacuum within the SAMs on Au TS determined from ARXPS (see Supplementary Fig. 6 for the XPS spectra) and molecular dynamics as a function of n , that is, the number of carbons under the Fc moiety (for details see Supplementary Methods : ‘Molecular Dynamics simulations: Model details and simulation protocol’). Error bars on the time- and structure-averaged MD data are 0.2–0.4 nm. ( f ) Cyclic voltammograms of SAMs of SC n FcC 13− n on Au with n =0, 3, 7, 10 and 13 (see Supplementary Figure 1 for cyclic voltammograms for all SAMs) recorded at a scan rate of 1.0 V s −1 with aqueous 1.0 M HClO 4 as the electrolyte solution. The peak oxidation potentials of the SAMs on Au TS generally increase with decreasing n suggesting the alkyl chains above the Fc units effectively shield the Fc units from the electrolyte solution. Full size image The molecule–electrode interaction To study the interaction of the Fc unit with the left electrode in more detail, we recorded ultraviolet photoelectron spectra (UPS) for the SAMs with small values of n on Ag TS and Au TS . The UPS data for SAMs on Ag and Au show similar trends; the UPS data for SAMs on Ag are discussed here and those for Au are shown in Supplementary Fig. 9 . 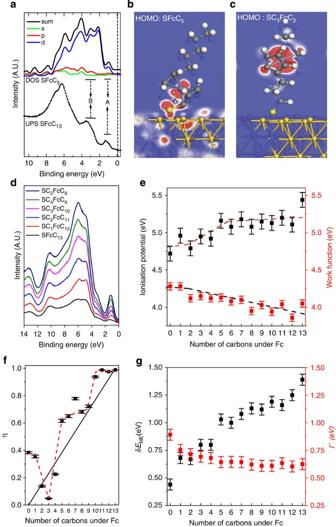Figure 4: Electronic structure of the SAMs on AuTSand AgTS. (a) The partial density of states (PDOS) calculated by DFT (seeSupplementary Fig. 11for all spectra) of SFcC5on Au and the experimental UPS data of SFcC13on AuTS. The two regions labelled with A and B indicate bands predominated by contributions from Fc and sulphur, respectively. The calculated structures of SFcC5(b) and SC3FcC2(c) on Au along with the charge density distribution of the HOMO. These calculations show that the HOMO is delocalized over the metal electrode for SFcC5on gold, while the HOMO is localized on the molecule and centred at the Fc unit for SC3FcC2on gold. SeeSupplementary Fig. 13for more details on the calculated charge distributions. (d) The UPS spectra for SCnFcC13−non AgTSwithn=0–5 (seeSupplementary Figs 9 and 10for all spectra, including on AuTS). (e) UPS measured work function and ionization potential (negative of the HOMO energy) values of the SCnFcC13−nSAMs on AgTSas a function of the number of carbons under the Fc units. The dashed lines are guides to the eye. Measured work functions are in excellent agreement with work functions computed from DFT electrostatic energy profiles (seeSupplementary Fig. 12). (f) The effective division parameterηVas calculated from the rectification data. The dashed line is a guide to the eye and the solid line represents the predicted values ofηVfor a linear electrostatic potential profile. (g) The width of the molecular orbital Γ and molecule–electrode offset energy δEMEas a function ofn. SeeSupplementary Discussionon ‘Valence band spectra’ for more details regarding the analysis and interpretation of the UPS data. Figure 4e shows that for SAMs with n >5, the HOMO energy level, E HOMO (eV), is nearly constant around −5.1±0.1 eV, but gradually increases to −4.7 eV as n decreases from 5 to 0. On the other hand, the work function of the Ag left electrode, Φ Ag (eV), gradually decreases from −4.0±0.1 eV to −4.3±0.1 eV as n decreases from 13 to 3, saturating at n <3. Hence, the value of δ E ME (= Φ Ag − E HOMO ) shows a noticeable decrease of ~0.5 eV as n decreases from 5 to 0 (as shown in Fig. 4g ). Figure 4: Electronic structure of the SAMs on Au TS and Ag TS . ( a ) The partial density of states (PDOS) calculated by DFT (see Supplementary Fig. 11 for all spectra) of SFcC 5 on Au and the experimental UPS data of SFcC 13 on Au TS . The two regions labelled with A and B indicate bands predominated by contributions from Fc and sulphur, respectively. The calculated structures of SFcC 5 ( b ) and SC 3 FcC 2 ( c ) on Au along with the charge density distribution of the HOMO. These calculations show that the HOMO is delocalized over the metal electrode for SFcC 5 on gold, while the HOMO is localized on the molecule and centred at the Fc unit for SC 3 FcC 2 on gold. See Supplementary Fig. 13 for more details on the calculated charge distributions. ( d ) The UPS spectra for SC n FcC 13− n on Ag TS with n =0–5 (see Supplementary Figs 9 and 10 for all spectra, including on Au TS ). ( e ) UPS measured work function and ionization potential (negative of the HOMO energy) values of the SC n FcC 13− n SAMs on Ag TS as a function of the number of carbons under the Fc units. The dashed lines are guides to the eye. Measured work functions are in excellent agreement with work functions computed from DFT electrostatic energy profiles (see Supplementary Fig. 12 ). ( f ) The effective division parameter η V as calculated from the rectification data. The dashed line is a guide to the eye and the solid line represents the predicted values of η V for a linear electrostatic potential profile. ( g ) The width of the molecular orbital Γ and molecule–electrode offset energy δ E ME as a function of n . See Supplementary Discussion on ‘Valence band spectra’ for more details regarding the analysis and interpretation of the UPS data. Full size image We performed density functional theory calculations (DFT; details are in Methods section) on a series of SC n FcC 5− n SAMs on Au with n from 0 to 5 to model the UPS spectra. The HOMO dominates the region just below the Fermi energy (labelled A in Fig. 4a ) and is associated with the Fc group and the thiolate sulphur bond to the bottom electrode ( Fig. 4b ). These calculations confirm that the HOMO is delocalized between the Fc orbital and the d-band of the metal surface via the sulphur binding group when n =0, or via both the sulphur binding group and the CH 2 units between the Fc when n =1 or 2. This hybridization explains the observed peak shifts and broadening in the UPS spectra [44] ( Fig. 4d,e ; see the Supplementary Discussion on ‘Valence band spectra’ for details). The DFT calculations ( Fig. 4 ) also show that the HOMO remains localized in the molecule when the Fc units and the sulphur are separated by three or more CH 2 units. Results from the full DFT data set are given in Supplementary Figs 11–13 . While molecule–electrode orbital hybridization can explain the shift of the HOMO level observed in the UPS spectra in the range of n =0–2, it does not account for the shifts over the entire range of n =3–5 of roughly 100–150 meV. The MD models indicate that a significant fraction of Fc units are within 5 Å of the Au surface for n =3–5, which is the critical distance for the H-atoms of the Fc units to form van der Waals contacts with the Au electrode [45] , as shown in Fig. 5c . We used dispersion-corrected DFT to estimate the strength of this interaction of the Fc units for various binding orientations of SC 3 Fc on Au(111) [46] , as described in detail in Supplementary Discussion : ‘Calculated Fc positions in the SAMs and van der Waals binding to the bottom electrode’. These calculations show that significant numbers of Fc units for n =3–5 do not couple to the Au electrode by direct Fc–Au chemisorption (in agreement with the UPS data), nor via the CH 2 units between the sulphur and the Fc unit, but interact instead via van der Waals Fc–electrode interactions with an estimated strength of 0.1–0.5 eV ( Fig. 5b ). 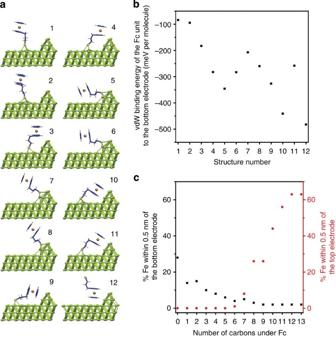Figure 5: Calculated Fc and electrode interactions and Fc positions. (a) SC3Fc molecule adsorption geometry on Au(111) (structures 1–12) computed using DFT. For details, seeSupplementary Discussion‘Fc---electrode van der Waal binding energies computed from Density Functional Theory (DFT) D3 calculations’. (b) Grimme D3 dispersion-corrected adsorption energies for Fc---Au(111) contacts in the 12 computed orientations. For reference, the MD van der Waals Fc---Au(111) binding energy averaged over all MD structures with Fc and Au distances ≤0.5 nm is 173±12 meV. (c) Populations of Fc units within 5 Å of the top and bottom electrode in SAM structures computed from molecular dynamics simulations. Figure 5: Calculated Fc and electrode interactions and Fc positions. ( a ) SC 3 Fc molecule adsorption geometry on Au(111) (structures 1–12) computed using DFT. For details, see Supplementary Discussion ‘Fc---electrode van der Waal binding energies computed from Density Functional Theory (DFT) D3 calculations’. ( b ) Grimme D3 dispersion-corrected adsorption energies for Fc---Au(111) contacts in the 12 computed orientations. For reference, the MD van der Waals Fc---Au(111) binding energy averaged over all MD structures with Fc and Au distances ≤0.5 nm is 173±12 meV. ( c ) Populations of Fc units within 5 Å of the top and bottom electrode in SAM structures computed from molecular dynamics simulations. Full size image We estimated the increase of the value of the energy coupling parameter Γ as a result of the Fc–electrode interaction from the experimental UPS data from the full width at half maximum (FWHM) of the peak in region A ( Fig. 4a ). The FWHM of peak A in the UPS data is nearly constant at ~0.62 eV for n =3–13 but rises to ~0.88 eV for n =0 ( Fig. 4g ). We note that in UPS the absolute value of FWHM depends on a number of factors including instrumental and spectral broadening, and screening effects, and therefore cannot provide reliable absolute values of Γ, but we believe that the relative increase in FWHM for low values of n gives a reasonable estimate for the increase in Γ caused by energy level broadening due to hybridization. The mechanism of rectification The shape of the electrostatic potential profile in a molecular junction has been thoroughly investigated theoretically [33] , [34] , [35] , [36] , [37] but has not been measured directly due to technical limitations. As discussed above, η V parameterises the electrostatic potential profile within the molecule on which R directly depends, among other factors (for example, level broadening, intrinsic coupling asymmetries, and so on). An empirical estimate of this parameter can be extracted from the experimental values of R as follows. The ratio between the potential drops at the left and right electrodes results in a rectification ratio R ∝ V R /V L (as described earlier). From the general definition of the voltage division parameter, η V ∝ V R /( V L +V R ), one can extract an effective value for η V from the rectification ratio as η V ∝ R/(R+ 1). This phenomenological relationship between η V and R can be used to extract a rough estimate of the shape of the potential drop profile in the junctions directly from the experimental data (see Fig. 4f ). We note that this method of determining the potential using R neglects the different nature of the couplings, for example, it does not account for level broadening which lowers R and results in an increase of η V for n <3, as described in the previous section. Figure 2e (and Fig. 4f ) shows that the transitions between the four coupling regimes are abrupt, and not gradual, and indicate that the electrostatic potential profile is more ramp-like (situations ii and iii), than flat (situation i), in character ( Fig. 1c ). In addition, Fig. 2f shows that the diodes are always in the ‘on-state’ and allow the current to pass through them at both directions of bias when n =5–9. The current across all junctions in the on-state are very similar ( Fig. 2f ) and therefore we believe that the mechanism of charge transport across these junctions is the same, based on sequential tunnelling (as described above and in reference [20] ). This observation implies that the electrostatic potential profile is not completely screened at the electrodes, and so the Fc units can still fall in between the energy window defined by the Fermi levels of both electrodes and participate in charge transport when bias is applied. The results demonstrate that the value of η V can be controlled as a function of the spatial position of the Fc units with respect to the electrodes, and that this relation is highly nonlinear. Although we cannot be quantitative, our experimental results suggest that the shape of the electrostatic potential profile resembles that of situation ii depicted in Fig. 1c , but further detailed (theoretical) investigations are needed to estimate the characteristic electric field screening length in this molecular junction, which we believe to be behind the observed nonlinear electrostatic potential profile. 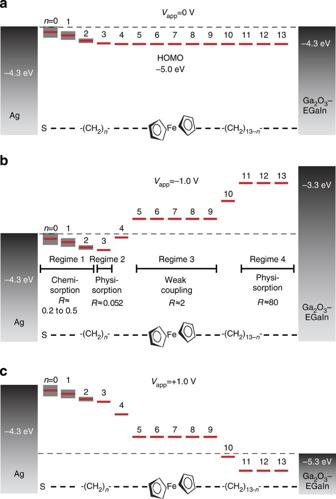Figure 6: The energy level diagrams of the diodes withn=0–13. The energy level diagrams are drawn for the junction under applied biases of 0 V (a), −1.0 V (b) and +1.0 V (c). The solid red markers indicate the position of the HOMO inside the junction and the number indicates the value ofn. For the values ofn=0–2, the grey box indicates the delocalization of the HOMO. The dashed grey line indicates the Fermi level of both electrodes at 0 V bias (top), Fermi level of the bottom electrode (left lead) at −1.0 V bias, and the Fermi level of the top electrode (right lead) at +1.0 V bias. In all of our experiments, we biased the Ga2O3/GaIn top electrode and grounded the Ag bottom electrode. Figure 6 shows the proposed energy level diagrams for the molecular diodes based on the results at 0 V ( Fig. 6a ), −1.0 V ( Fig. 6b ) and +1.0 V ( Fig. 6c ) applied bias. This figure illustrates the 14 different positions of the HOMO inside the junctions as a function of n and the four distinct Fc–electrode coupling regimes revealed by the data. Regime 1 is the range in which the close proximity of the Fc to the left electrode ( n <3) results in hybridization of the HOMO with the metal–electrode and large values of Γ, which makes δ E ME <Γ, resulting in large leakage currents. The junctions do not rectify even though the condition η V ≪ ½ is met. In Regime 2, the non-covalent coupling of the Fc (0.1–0.5 eV) to the bottom electrode ( n =3 and 4) results in narrow molecular energy levels (low Γ), making δ E ME ≈Γ. This larger δ E ME /Γ ratio reduces leakage currents and the junctions rectify with η V close to zero and R =0.052. For Regime 3, the weak coupling of the Fc to both electrodes ( n =5–9) together with a nonlinear electrostatic potential profile along the molecule (that is, η V is ~½) results in diodes that are in the on-state in both directions of bias, resulting in low values of R ( Fig. 2e ). In Regime 4, the non-covalent coupling of the Fc to the top electrode for n =11–13 results in optimal values of Γ (that is, sufficiently large δ E ME /Γ ratios) and large rectification ratios (with η V ~1). We do not know the δ E ME values of the HOMO level with the right electrode, but we expect Γ to be substantially smaller based on the much higher rectification ratio ( R ~80) for junctions with n >10. Figure 6: The energy level diagrams of the diodes with n =0–13. The energy level diagrams are drawn for the junction under applied biases of 0 V ( a ), −1.0 V ( b ) and +1.0 V ( c ). The solid red markers indicate the position of the HOMO inside the junction and the number indicates the value of n . For the values of n =0–2, the grey box indicates the delocalization of the HOMO. The dashed grey line indicates the Fermi level of both electrodes at 0 V bias (top), Fermi level of the bottom electrode (left lead) at −1.0 V bias, and the Fermi level of the top electrode (right lead) at +1.0 V bias. In all of our experiments, we biased the Ga 2 O 3 /GaIn top electrode and grounded the Ag bottom electrode. Full size image The best balance between molecule–electrode offset energy δ E ME , asymmetry parameter η V and molecular orbital width Γ, resulting in a large rectification ratio, is achieved when the ferrocenyl-centred HOMO is coupled to one of the electrodes via non-covalent interactions (physisorption), rather than via strong chemical interactions (chemisorption). Three CH 2 units are required experimentally to avoid molecular level broadening through the thiolate anchoring group. On the other hand, four to five CH 2 units are required experimentally to position the Fc units sufficiently far away from either electrode to switch off rectification. By gradually shifting the position of the Fc units from the top to bottom of the SAM, we controlled the direction of rectification and estimate crudely the nonlinear shape of the electrostatic potential profile of the junctions. More comprehensive experimental and theoretical experiments are needed to improve the understanding of the mechanism of charge transport and how, for instance, the molecules screen the electric fields or to elucidate the details of the mechanism of the sequential tunnelling process [47] , [48] . In general, the active components of molecular electronic devices may interact with metal ad-atoms or couple to the electrodes via other mechanisms, such as, induced density of interface states or metal-induced gap states [49] , [50] , which can also extend up to three CH 2 units into the SAMs. Therefore, we believe that our experimentally established ‘design rules’ to fine-tune the coupling of molecular orbitals with the electrodes are particularly important for the rational design of molecular electronic devices, and are broadly applicable to other devices where metal– or semiconductor–organic interfaces have a key role, ranging from organic solar cells and light-emitting diodes to biomolecular devices [51] , [52] . Metal evaporation We prepared Ag and Au surfaces for the formation of SAMs by evaporation of silver and gold on silicon wafers (100, p-type) by electron-beam (e-beam) evaporation (Edwards, Auto 306). The metal we used had a purity of 99.999% as obtained from Super Conductor Materials, Inc (USA). The e-beam evaporator was operated at a base pressure of ~2 × 10 −6 bar to deposit a layer of 500 nm of Ag or Au using a deposition rate for the first 50 nm of 0.3–0.5 Å s −1 and the remaining 450 nm at a rate of 1 Å s −1 . Sample preparation The synthesis of all ferrocenyl derivatives is described in Supplementary Methods : ‘Synthesis of n-alkanethiols with Fc group (HSC n FcC 13− n ; n = 0–13)’. The formation of SAMs and the preparation of the template-stripped Au and Ag surfaces used in this study followed our reported procedure [27] . Briefly, we cleaned glass slides of dimension 1 × 1 cm 2 (7,105 microscope slide, 1 mm thick) by immersion in a solution of H 2 SO 4 : H 2 O 2 : H 2 O=1: 1: 5 at 70 °C for 20 min, followed by rinsing of the substrates with deionized water after which the slides were blown to dryness in a stream of N 2 gas. These glass slides were further cleaned in a plasma of O 2 for 5 min at 500 mTorr. We used the optical adhesive (Norland, No. 61) to glue the glass slides on to the as-deposited Ag/Au surfaces on Si/SiO 2 . The substrates were placed under ultraviolet light for 1 h using a light source of 100 Watt to cure the optical adhesive. Before the formation of the SAMs, we used a razor blade to cut the sides of the glass and then cleave off the metal surface from the Si wafer. Within ~5 s, we immersed these surfaces in 3 mM ethanolic solutions of the HSC n FcC 13− n to minimize contamination of the surfaces from the ambient. The SAMs were formed over a period of time of 3–6 h at room temperature, and then were rinsed gently by EtOH and dried in a stream of N 2 gas. Electrochemistry The SAMs of SC n FcC 13− n on Au TS electrodes were electrochemically characterized using cyclic voltammetry performed with an AUTOLAB PGSTAT302N with NOVA 1.9 software. A custom-built electrochemical cell was equipped with a Pt-disk counter electrode, Ag/AgCl reference electrode and the Au TS working electrode area exposed to the HClO 4 electrolyte solution was 0.33 cm 2 . We placed this electrochemical cell in a Faraday cage and recorded cyclic voltammograms of the SAMs in an aqueous solution of 1.0 M HClO 4 at a scan rate of 1.0 V s −1 in the range −0.1 to +0.9 V. Synchrotron radiation-based spectroscopy measurements Synchrotron-based photoemission spectroscopy (PES) and NEXAFS measurements were carried out at the SINS (Surface, Interface and Nanostructure Science) beamline of Singapore Synchrotron Light Source. All the measurements were performed at room temperature in an ultrahigh vacuum chamber with a base pressure of 1 × 10 −10 mbar (ref. 53 ). The photon energy was calibrated using the Au 4 f 7/2 core level peak at 84.0 eV of a sputter-cleaned gold foil in electrical contact with the sample. All the PES spectra are normalized by the photon current. The work function was measured using 60 eV photon energy and −9 V bias was applied to the sample to overcome the work function of the analyser. Photon energy values of 850, 350 and 60 eV were used to probe the Fe 2 p 3/2 , S 2 p and valence band spectra, respectively. The least-square peak fit analysis was performed using XPSpeak software. The sloping background was modelled using Shirley plus linear background correction and the photoemission profiles with Voigt functions (Lorentzian (30%) and Gaussian (70%)). For S 2 p spectra fitting, a splitting difference of ~1.18 eV and branching ratio of 2 (2 p 3/2 ): 1 (2 p 1/2 ) were used [54] . The high-resolution PES spectra of Fe 2 p 3/2 and S 2 p of SC n FcC 13− n SAMs on Au TS are shown in Supplementary Fig. 6 and their relative intensity summarized in Supplementary Table 3 . Angular-dependent C K -edge NEXAFS spectra were collected in Auger electron yield mode using a Scienta R4000 electron energy analyser. The linear polarization factor of the X-ray beam was measured to be >90%. The photon energy of the incident X-ray was calibrated using sputter-cleaned gold foil. All SAM NEXAFS spectra were first normalized relative to the clean-metal NEXAFS spectrum. Furthermore, the spectra were normalized to have the same absorption edge jump between 280 and 320 eV. The junction measurements by EGaIn technique We used cone-shaped tips of Ga 2 O 3 /EGaIn as top electrodes using a previously described home-built system [27] . This technique makes it possible to form junctions in which the electrical characteristics are dominated by the chemical and supramolecular structure of the SAMs inside the junctions and to record data with statistically large numbers [20] . Device properties are not dominated by any of the other asymmetries, nor by the Ga 2 O 3 layer, present in these junctions [26] . Statistical analysis The junctions of each type of SAM were fabricated on three different Ag TS samples using the ‘EGaIn-technique’. We formed six to eight junctions on each substrate. For each junction, we recorded 24 scans (0 V→−1.0 V→1.0 V and back to 0 V) with a 50-mV step and 0.2-s delay. We collected more than 500 traces for each type of SAM (see Supplementary Table 2 ), and we calculated log | J | and log R using previously reported methods [55] . Supplementary Figure 4 shows that the log-average J (V) curves and the error bars represent the one log-standard deviations. Supplementary Figure 5 shows the histograms of the values of R measured at ±1.0 V with Gaussian fits to these histograms that we used to determine the log-average values of R and their log-standard deviations are listed in Supplementary Table 2 . Molecular simulations Density of states (DOS) distributions were calculated from DFT band structures and compared with UPS spectra. Molecular dynamics simulations were used to calculate the structure, dynamics and energetics of 1,216-molecule SAMs on silver and gold, and were supplemented with dispersion-corrected DFT calculations [46] to estimate Fc---metal interaction strengths. DFT calculations were also used to calculate work function shifts on SAM-covered electrode surfaces and compare with UPS measurements. Brief summaries are given below of the computational models and methods used. Further details of the simulations are provided in Supplementary Methods ‘Molecular Dynamics simulations: Model details and simulation protocol’ and Supplementary Discussion ‘Fc---electrode van der Waal binding energies computed from Density Functional Theory (DFT) D3 calculations’ and ‘Work function shifts calculated from Density Functional Theory’, as well as Supplementary Fig. 17 and 18 . All simulation files and computed structures are available on request from the corresponding authors. Density functional theory (DFT) band structure calculations were performed using the CASTEP package with ultra-soft pseudopotentials and a 280-eV cut-off energy [56] , [57] . A plane wave basis set was used, and the exchange-correlation was treated with the generalized gradient approximation GGA [58] . DOS was calculated by integrating over the Brillouin zone using a 3 × 3 × 1 k-point sampling grid. The gold surface was simulated using a three-layer bulk terminated slab with static gold atoms. In all simulations, a p (3 × 3) unit cell was used, which corresponds to a surface coverage of 2.2 × 10 −10 mol cm −2 . The slab was repeated periodically with 35 Å of vacuum between the slabs in the direction normal to the surface plane. For the structure optimization, we used the Perdew, Burke and Ernzerhof PBE exchange-correlation functional [59] . To describe the configuration of the SC n FcC 5− n on Au (111), the molecules were relaxated using the BFGS algorithm [60] and bonding of the molecules to the surface was described using the DOS distribution to quantify the adsorbate–substrate electronic interaction. A partial DOS analysis is used to describe the different electronic interactions between the molecule and the surface as the Fc moiety is positioned progressively further away from the surface, that is, as n in SC n FcC 5− n is increased from 0 to 5. A slab of silver surface Ag(111) of area 33 nm × 13 nm, or 429 sq nm, was cut from bulk silver metal and 1,216 ferrocene–alkanethiol molecules were placed on one face with an initial density of 4.5 × 10 −10 mol cm −2 to match the maximum surface coverage measured by cyclic voltammetry ( Supplementary Table 1 ). Calculations were performed using the NAMD program [61] with the CHARMM force field [45] . Statistics were generated from the final 2 ns of 17 ns of dynamics for each model, sampling every 20 ps to provide 100 statistically independent structures for each SAM. The structure formed for the SAM with n =9 is shown in Supplementary Fig. 14 . In all, 221 ns of dynamics were performed on the 13 different SC n FcC 13− n SAMs with n =0–12. The SAMs formed from the molecule with Fc at the top of the alkyl chain, SC 13 Fc, were modelled using the same protocol in earlier work [30] . Control simulations of SAM chemisorption on Au required an additional 65 ns of dynamics (5 ns of production dynamics for each SAM with a target Au–S–C bond angle of 109°) [45] . All data points and error bars reported were calculated over ~25,000 molecule conformations for each SAM (a central ~250-molecule sampling disk sampled 100 times). Image generation and Tcl script-based trajectory analysis was performed using the VMD program. [62] How to cite this article: Yuan, L. et al . Controlling the direction of rectification in a molecular diode. Nat. Commun. 6:6324 doi: 10.1038/ncomms7324 (2015).